Cell cycle transition from S-phase to G1 inCaulobacteris mediated by ancestral virulence regulators Zinc-finger domain transcriptional regulators regulate a myriad of functions in eukaryotes. Interestingly, ancestral versions (MucR) from Alpha-proteobacteria control bacterial virulence/symbiosis. Whether virulence regulators can also control cell cycle transcription is unknown. Here we report that MucR proteins implement a hitherto elusive primordial S→G1 transcriptional switch. After charting G1-specific promoters in the cell cycle model Caulobacter crescentus by comparative ChIP-seq, we use one such promoter as genetic proxy to unearth two MucR paralogs, MucR1/2, as constituents of a quadripartite and homeostatic regulatory module directing the S→G1 transcriptional switch. Surprisingly, MucR orthologues that regulate virulence and symbiosis gene transcription in Brucella , Agrobacterium or Sinorhizobium support this S→G1 switch in Caulobacter . Pan-genomic ChIP-seq analyses in Sinorhizobium and Caulobacter show that this module indeed targets orthologous genes. We propose that MucR proteins and possibly other virulence regulators primarily control bacterial cell cycle (G1-phase) transcription, rendering expression of target (virulence) genes periodic and in tune with the cell cycle. How S-phase cells instate the G1-phase transcriptional programme is poorly understood. The synchronizable Alpha-proteobacterium Caulobacter crescentus (henceforth Caulobacter ) is the pre-eminent model system commonly used to dissect cell cycle transcription at the most fundamental level [1] , [2] . Caulobacter divides into a smaller and motile swarmer cell and a larger and sessile stalked cell, residing in G1- and S-phase, respectively ( Fig. 1a ). Such asymmetric division has also been reported for related Alpha-proteobacterial pathogens/symbionts [3] belonging to the genera Brucella , Agrobacterium or Sinorhizobium, some of which are also synchronizable [4] , [5] . As Alpha-proteobacteria generally encode most known cell cycle regulatory proteins originally identified in Caulobacter [6] , the underlying mechanisms for the G1-phase transcriptional programme seem to be conserved and perhaps serve to control expression of virulence/symbiosis functions as a function of the cell cycle. Indeed, virulence functions are typically present in non-replicative dispersal cell types of unrelated pathogens such as members of the Chlamydiae [7] , and features of an underlying cytological and/or molecular asymmetry have also been reported for the pathogenic Gamma-proteobacteria Pseudomonas aeruginosa and Klebsiella pneumoniae [8] and distantly related mycobacteria [9] . This suggests that the implementation of daughter cell-specific transcriptional programs is pervasive among different prokaryotic lineages, and that lineage-specific mechanisms direct this re-programming. 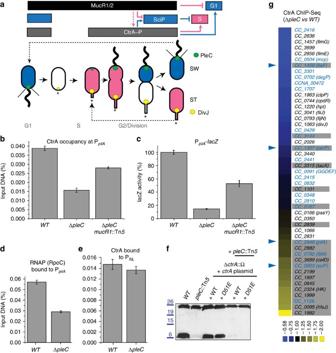Figure 1: CtrA-bound promoters that are affected in ΔpleCcells. (a) Schematic of the regulatory interactions betweenctrA,sciPandmucR1andmucR2 (mucR1/2)during theC. crescentuscell cycle. Phosphorylated CtrA (CtrA~P) activates transcription of S- and G1-phase genes. In S-phase, MucR1/2 represses G1-genes such assciP. ThesciPgene is activated in G1 and the newly synthesized SciP translation product represses S-phase promoters. The antagonistic kinase/phosphatase pair, DivJ (yellow dot) and PleC (green dot) indirectly influence CtrA~P and partition with the stalked (ST) cell chamber or swarmer (SW) cell chamber, respectively. PleC promotes CtrA~P accumulation in the SW cell. The dashed arrow indicates that MucR1/2 promote expression of CtrA, but not necessarily its phosphorylation. The star denotes the holdfast. Blue colouring denotes G1-phase transcription, whereas pink is for the late S-phase programme. Light grey labels indicate the cell cycle stages. (b–e) Occupancy of CtrA and RNA polymerase (RNAP) at thepilA(PpilA) andfliLpromoter (PfliL)) inWT(NA1000), ΔpleCand ΔpleC mucR1::Tn5mutant cells as determined by quantitative chromatin immunoprecipitation assays (qChIP) using antibodies to CtrA or RpoC, as well aspilAtranscription measurements conducted using a PpilA-lacZpromoter-probe reporter. Data are from three biological replicates. Error is shown as s.d. (f) Immunoblots showing PilA (lower band, approximately 6 kDa) and CtrA (upper band, approximately 26 kDa) steady-state levels inWTandpleC::Tn5mutant cells harbouringWT ctrAor phosphomimeticctrA(D51E)expressed from a plasmid in the absence of chromosomally encoded CtrA (ΔctrA::Ω). Molecular size standards are indicated on the left as blue lines with the corresponding values (blue) in kDa. (g) Comparative ChIP-seq performed with antibodies to CtrA on chromatin fromWTand ΔpleCcells. Boxed in grey are PleC:CtrA promoters that were verified as being PleC dependent (Supplementary Fig. 1B). Blue labels indicate PleC:CtrA promoters that are bound by MucR1/2 as determined by the ChIP-seq experiments (Fig. 2). Blue arrowheads point to promoters for which the ChIP-seq traces are shown inFig. 5. The colour key at the bottom indicates the degree by which the occupancy of CtrA is altered by the ΔpleCmutation, expressed as log2ratio (Supplementary Data 1). Figure 1: CtrA-bound promoters that are affected in Δ pleC cells. ( a ) Schematic of the regulatory interactions between ctrA , sciP and mucR1 and mucR2 (mucR1/2) during the C. crescentus cell cycle. Phosphorylated CtrA (CtrA~P) activates transcription of S- and G1-phase genes. In S-phase, MucR1/2 represses G1-genes such as sciP . The sciP gene is activated in G1 and the newly synthesized SciP translation product represses S-phase promoters. The antagonistic kinase/phosphatase pair, DivJ (yellow dot) and PleC (green dot) indirectly influence CtrA~P and partition with the stalked (ST) cell chamber or swarmer (SW) cell chamber, respectively. PleC promotes CtrA~P accumulation in the SW cell. The dashed arrow indicates that MucR1/2 promote expression of CtrA, but not necessarily its phosphorylation. The star denotes the holdfast. Blue colouring denotes G1-phase transcription, whereas pink is for the late S-phase programme. Light grey labels indicate the cell cycle stages. ( b – e ) Occupancy of CtrA and RNA polymerase (RNAP) at the pilA (P pilA ) and fliL promoter (P fliL) ) in WT (NA1000), Δ pleC and Δ pleC mucR1 ::Tn 5 mutant cells as determined by quantitative chromatin immunoprecipitation assays (qChIP) using antibodies to CtrA or RpoC, as well as pilA transcription measurements conducted using a P pilA - lacZ promoter-probe reporter. Data are from three biological replicates. Error is shown as s.d. ( f ) Immunoblots showing PilA (lower band, approximately 6 kDa) and CtrA (upper band, approximately 26 kDa) steady-state levels in WT and pleC ::Tn 5 mutant cells harbouring WT ctrA or phosphomimetic ctrA(D51E) expressed from a plasmid in the absence of chromosomally encoded CtrA (Δ ctrA ::Ω). Molecular size standards are indicated on the left as blue lines with the corresponding values (blue) in kDa. ( g ) Comparative ChIP-seq performed with antibodies to CtrA on chromatin from WT and Δ pleC cells. Boxed in grey are PleC:CtrA promoters that were verified as being PleC dependent ( Supplementary Fig. 1B ). Blue labels indicate PleC:CtrA promoters that are bound by MucR1/2 as determined by the ChIP-seq experiments ( Fig. 2 ). Blue arrowheads point to promoters for which the ChIP-seq traces are shown in Fig. 5 . The colour key at the bottom indicates the degree by which the occupancy of CtrA is altered by the Δ pleC mutation, expressed as log 2 ratio ( Supplementary Data 1 ). Full size image In Caulobacter , the two daughter cell types can be conveniently discerned based on functional and morphological criteria: while the G1-phase cell harbours several adhesive pili and a single flagellar motor at the old pole, the S-phase cell harbours a stalk with an adhesive holdfast at the corresponding pole. In addition, these two cell types differ in their buoyancy, a feature that is exploited for the enrichment of a pure population of G1 cells on a density gradient [10] . A hallmark of the Caulobacter G1→S transition is the loss of the flagellum and pili, the elaboration of a stalk and holdfast, as well as the switch in cellular buoyancy. In the ensuing S-phase, cells segregate the replicated DNA, activate motility genes and assemble the flagellar motor and pilus secretion apparatus at the pole opposite the stalk [1] . As soon as the pre-divisional cell compartmentalizes, the G1-phase transcriptional programme is instated in the swarmer chamber, pili are extruded, the flagellum is energized and the cellular buoyancy is reversed. In the stalked chamber, DNA replication re-initiates and S-phase transcription resumes. How the switch from S-phase to the G1-phase transcriptional programme (henceforth referred to as S→G1 transcriptional switch) is induced at compartmentalization is unresolved. P pilA , the promoter of the gene encoding the structural component of the pilus filament ( pilA) , is a target of this regulation and thus suitable as genetic proxy. P pilA is activated in G1-phase [11] by the conserved and essential cell cycle transcriptional regulator A (CtrA) [12] . CtrA can function either as activator or repressor of transcription and also as an inhibitor of DNA replication by directly binding the TTAA-N(7)-TTAA target motif (CtrA box) in promoters and the origin of replication, Cori [1] . Binding of CtrA to its targets is enhanced by phosphorylation (CtrA~P) of aspartate 51 (D51) by way of a complex phosphorelay involving the conserved and essential hybrid histidine kinase CckA [13] . CtrA is proteolytically removed during the G1→S transition, re-synthesized and again proteolysed by the ClpXP protease in the nascent S-phase chamber upon compartmentalization [1] ( Fig. 1a ). Thus, CtrA is not a G1-specific regulator as it is already present and active before compartmentalization (that is, in late S-phase), for example, at promoters of early (class II) flagellar and other motility genes [1] , [14] . Determinants other than CtrA~P likely promote the switch from S→G1 phase transcription of CtrA-dependent genes during compartmentalization [15] , [16] . A candidate for such an accessory role is the conserved helix-turn-helix motif protein SciP that accumulates in G1-phase [17] , [18] . SciP binds CtrA directly and impairs CtrA’s ability to recruit RNA polymerase (RNAP) holoenzyme to P pilA and other CtrA-activated promoters in vitro , apparently without establishing sequence-specific contacts to DNA [18] , [19] . An alternative view holds that SciP does not require CtrA to bind DNA. Instead, SciP was proposed to bind DNA directly at the 5′-TGTCGCG-3′ motif in the ctrA promoter in vitro [17] . Surprisingly, the occurrence of this motif (>1,460 predicted sites in the 4.01 Mbp GC-rich Caulobacter genome) vastly exceeds the number of previously predicted CtrA target promoters with 1–4 CtrA boxes (~50) [1] . Also, mutation of the 5′-TGTCGCG-3′ motif did not affect binding of CtrA and SciP to P pilA in vitro [19] . As both models posit that SciP targets all CtrA-dependent promoters, further investigations on the S→G1 transcriptional switch and on the possible role of SciP in this event are warranted. Here we report a system-level and forward genetic approach for the dissection of this transcriptional switch. We unearth two uncharacterized ancestral zinc-finger domain proteins, MucR1 and MucR2, as key determinants of a novel quadripartite and homeostatic regulatory module that together with CtrA and SciP turn on G1-phase genes and concomitantly shut off S-phase genes, respectively. Using pan-genomic ChIP-seq (chromatin immunoprecipitation coupled to deep-sequencing), we reveal MucR as a direct regulator of orthologous genes in Sinorhizobium that can direct cell cycle transcription in Caulobacter . Thus, a conserved genetic module uses an ancestral transcription factor fold, extensively researched in the eukaryotic domain of life [20] , to integrate virulence, symbiosis and/or cell cycle transcription in a bacterial lineage from which eukaryotic organelles descended [21] . Target promoters of the S→G1 transcriptional switch Before surveying the extent of the S→G1 promoter switch on a genome-wide scale, we first characterized candidate promoters by quantitative ChIP (qChIP) following precipitation with polyclonal antibodies to CtrA and monoclonal antibodies to the RpoC (β′) subunit of RNAP from chromatin of wild-type ( WT ) and Δ pleC cells. pleC encodes a histidine kinase/phosphatase that partitions with the G1-phase progeny ( Fig. 1a ) and is required for the accumulation of G1-specific transcripts, including pilA , and for maximal accumulation of CtrA~P [15] . qChIP confirmed that CtrA and RNAP occupancy at P pilA are 58 and 48% less abundant in Δ pleC cells compared with WT cells ( Fig. 1b ), consistent with the reduced P pilA activity ( Fig. 1b–d ). We also noted a similar reduction in CtrA occupancy at P tacA, (the promoter of the G1-phase gene tacA ), along with a commensurate reduction in promoter activity (as determined using the P tacA - lacZ promoter-probe reporter, Supplementary Fig. 1A ). By contrast, CtrA abundance at P fliL (the promoter of the class II flagellar gene fliL ) was not noticeably affected ( Fig. 1e ). Knowing that fliL mRNA peaks in late S-phase (~84 min), that the pilA and tacA mRNAs surge in G1 (~120 min (ref. 16 )) and that PilA accumulation is PleC-dependent ( Fig. 1f ), we hypothesized that PleC-dependent CtrA (PleC:CtrA) target promoters regulate G1-phase genes. Next, we charted other PleC:CtrA target promoters on a genome-wide scale by comparative ChIP-seq of CtrA occupancy in WT and Δ pleC cells. Bioinformatic analyses predicted >100 CtrA target sites that, akin to P pilA , are bound substantially less efficiently by CtrA (that is, with log 2 difference of <−0.8) in Δ pleC versus WT cells ( Figs 1g and 2a ; and Supplementary Data 1 ). To confirm that these sites indeed harbour PleC:CtrA target promoters, we constructed promoter-probe reporters of the top 18 PleC:CtrA target sites and measured promoter activities in WT and Δ pleC cells ( Supplementary Figs 1B and 2A,B ). All reporters were less active in Δ pleC cells, showing that they indeed harbour PleC:CtrA target promoters. Since the transcripts produced from these promoters are restricted to G1-phase [15] , [22] , we conclude that these sites define a new class of G1-phase promoters that are activated by CtrA in a PleC-dependent manner. Importantly, the promoter of the G1-phase gene sciP (P sciP ) also falls into this class ( Supplementary Fig. 1B ; see below). 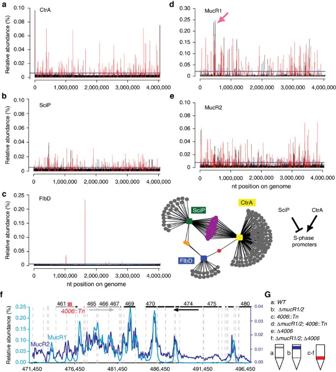Figure 2: Genome-wide occupancy of CtrA, SciP, FlbD, MucR1 and MucR2. (a–e). Genome-wide occupancies of CtrA (a), SciP (b), FlbD (c), MucR1 (d) and MucR2 (e) on theC. crescentusgenome as determined by ChIP-seq. Note that owing to the ability of the anti-MucR2 antibody to precipitate MucR1, some of the peaks inecould also derive from MucR1, but this is also expected as we show inFig. 4athat MucR1 can interact with MucR2. Thexaxis represents the nucleotide position on the genome, whereas theyaxis denotes the relative abundance of reads for each probe (seeSupplementary Methodsfor detailed description). Candidate peaks reported in each profile are shown as red bars (‘ANNO probes’;Supplementary Data 1–5), whereas a horizontal blue line in each profile denotes the cutoff applied to separate peaks and background. The middle panel incdepicts the minimal overlap between the targets of SciP, CtrA and FlbD, whereas the right panel illustrates the regulatory relationship between SciP, CtrA and S-phase promoters. The pink arrow inddenotes the 26-kb mobile genetic element (MGE) enlarged inf. (f) ChIP-seq trace of MucR1 (light blue) and MucR2 (dark blue) on the 26-kb MGE. Genes encoded from right to left are shown in grey bars, whereas the black bars indicate genes on the reverse strand. The numbers above refer to the CCNA gene annotation. Thehimar1(Tn) insertions inCCNA_04006are shown as vertical red bars. (g) Buoyancy ofWT(grey) and mutant (blue or red) cells harbouring ahimar1(Tn) insertion or an in-frame deletion (Δ) inCCNA_04006(4006). The schematic shows the sedimentation of cells after Percoll density gradient centrifugation in a test tube. AlthoughWTcells show the typical upper and lower buoyancy conferred by S and G1 cells, respectively, ΔmucR1/2cells only show the former.CCNA_04006is epistatic overmucR1/2,as inactivationCCNA_04006confers the latter buoyancy. Figure 2: Genome-wide occupancy of CtrA, SciP, FlbD, MucR1 and MucR2. ( a – e ). Genome-wide occupancies of CtrA ( a ), SciP ( b ), FlbD ( c ), MucR1 ( d ) and MucR2 ( e ) on the C. crescentus genome as determined by ChIP-seq. Note that owing to the ability of the anti-MucR2 antibody to precipitate MucR1, some of the peaks in e could also derive from MucR1, but this is also expected as we show in Fig. 4a that MucR1 can interact with MucR2. The x axis represents the nucleotide position on the genome, whereas the y axis denotes the relative abundance of reads for each probe (see Supplementary Methods for detailed description). Candidate peaks reported in each profile are shown as red bars (‘ANNO probes’; Supplementary Data 1–5 ), whereas a horizontal blue line in each profile denotes the cutoff applied to separate peaks and background. The middle panel in c depicts the minimal overlap between the targets of SciP, CtrA and FlbD, whereas the right panel illustrates the regulatory relationship between SciP, CtrA and S-phase promoters. The pink arrow in d denotes the 26-kb mobile genetic element (MGE) enlarged in f . ( f ) ChIP-seq trace of MucR1 (light blue) and MucR2 (dark blue) on the 26-kb MGE. Genes encoded from right to left are shown in grey bars, whereas the black bars indicate genes on the reverse strand. The numbers above refer to the CCNA gene annotation. The himar1 ( Tn ) insertions in CCNA_04006 are shown as vertical red bars. ( g ) Buoyancy of WT (grey) and mutant (blue or red) cells harbouring a himar1 ( Tn ) insertion or an in-frame deletion (Δ) in CCNA_04006 ( 4006 ). The schematic shows the sedimentation of cells after Percoll density gradient centrifugation in a test tube. Although WT cells show the typical upper and lower buoyancy conferred by S and G1 cells, respectively, Δ mucR1/2 cells only show the former. CCNA_04006 is epistatic over mucR1/2, as inactivation CCNA_04006 confers the latter buoyancy. Full size image SciP preferentially binds S-phase target promoters of CtrA ChIP-seq experiments ( Fig. 2b ) with a polyclonal antibody to SciP revealed that SciP does not associate with all CtrA target sites ( Fig. 2a ) in vivo . In fact, we observed a clear promoter preference for SciP, targeting the S-phase promoters, but not G1-phase promoters activated by CtrA. Bioinformatic analyses predicted 76 SciP-binding sites in vivo (see Methods section and Supplementary Data 2 ) upstream of CtrA-activated genes whose transcripts all peak in late S-phase [16] , such as flagellar genes (for example, flmG , pleA , fliQ , fliX , flgB , fliL , fliI and fljJ ), pilus secretion genes (for example, cpaB and others, see below) and chemotaxis gene orthologues (for example, CC_2317 , CC_2281 and CC_1655 ). If SciP binds DNA only through a direct association with CtrA, then all CtrA targets, including Cori and CtrA-repressed promoters, should be efficiently precipitated with the SciP antibody. These CtrA target sites as well as those of PleC:CtrA (G1) promoters such as P pilA were not enriched in the ChIP sample, indicating that they are not preferred targets of SciP in vivo ( Supplementary Discussion ). A MEME-based motif search using 50 of the top SciP target sites predicted 5′-(G/A) TTAA CCAT(A/G)-3′ as possible SciP consensus motif ( Supplementary Data 2 ), a motif having half a CtrA box (underlined, see above) and often overlapping with the CtrA target site in promoters ( Supplementary Data 2 ). These results suggest that CtrA and SciP compete for binding to these promoters, or that repression by SciP involves a cooperative binding mode between SciP and CtrA at this site, perhaps through an ‘extended’ CtrA box that includes a CtrA half site harbouring a SciP consensus motif. Interestingly, combinatorial promoter control by two regulators has been described during sporulation in the unrelated Delta-proteobacterium Myxococcus xanthus [23] . Our results also reveal that SciP binds neither P fliF (the promoter of the class II flagellar gene fliF that is activated by CtrA in S-phase [16] ) nor P pilA efficiently in vivo . We therefore suggest that the ability of SciP to interfere with the recruitment of RNAP to CtrA~P-activated promoters such as P fliF and P pilA in vitro [18] , [19] likely reflects a secondary, later-acting mechanism to silence CtrA-dependent transcription. It is conceivable that this mechanism comes into play later in G1-phase once CtrA activated transcription of sciP and other genes (that is, after compartmentalization) has led to a build-up of a threshold in SciP. Since our ChIP-seq experiments failed to reveal SciP at all CtrA-activated promoters, it seems that SciP binds the bipartite CtrA target complex weakly and/or only very transiently in vivo . The simplest interpretation of our ChIP-seq data is that SciP stably associates with promoters that CtrA activates in S-phase, while promoters that CtrA activates in G1-phase or represses (such as the podJ or ftsZ promoter) are not preferred targets of SciP in vivo . SciP also does not target the CtrA-bound Cori site or the CtrA-activated promoter P fliF efficiently in vivo . P fliF is repressed by FlbD, the σ 54 -dependent transcriptional activator of class III/IV and repressor of class II flagellar promoters [14] . Our ChIP-seq experiments showed that FlbD binds P fliF and several other class III/IV flagellar promoters ( Fig. 2c and Supplementary Fig. 3 ). FlbD also targets, in a mutually exclusive fashion with SciP, class II flagellar promoters ( Fig. 2c and Supplementary Discussion ), but neither P pilA nor other PleC:CtrA target promoters. MucR1/2 binds promoters of G1-phase genes Our observation that phosphomimetic variants of CtrA cannot elevate P pilA activity in Δ pleC cells ( Supplementary Fig. 1C ) and PilA protein accumulation, regardless of whether WT CtrA is present or not ( Fig. 1f ), predicted an unknown repressor(s) that prevents CtrA-mediated activation at P pilA , P sciP and other G1-promoters in Δ pleC cells. To identify this repressor, we mutagenized Δ pleC cells harbouring a P pilA - nptII transcriptional reporter (integrated at the chromosomal pilA locus; pilA ::P pilA - nptII ) with a mini-Tn 5- Gm R (encoding gentamycin resistance, Gm R ). Selecting for kanamycin-resistant transposon mutants in which P pilA - nptII expression had been restored ( Fig. 3a ), we isolated one such mutant ( mucR1 ::Tn 5 ) and determined the Tn 5 insertion to be in the middle (codon 74) of the mucR -like gene CC_0933 ( CCNA_00982 , henceforth mucR1 ; Supplementary Fig. 1D ). MucR1 belongs to the conserved MucR/Ros family of transcriptional regulators that harbour a zinc-finger-type fold [24] and control virulence, symbiosis and/or motility in the human pathogen Brucella suis [25] , the plant pathogen Agrobacterium tumefaciens [26] and the plant symbiont Sinorhizobium fredii NGR234 (ref. 24 ). 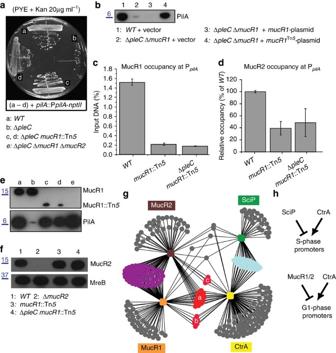Figure 3: Identification ofmucR1/2as negative regulator of PleC:CtrA promoters. (a) Growth ofWT(a) ΔpleC(b) and derivatives (c,d) carrying thepilA::PpilA–nptIItranscriptional reporter on PYE plates containing kanamycin (20μg ml−1). (b) Immunoblot showing PilA steady-state levels inWTand ΔpleCΔmucR1double-mutant cells harbouring the empty vector (1 and 2, respectively), and ΔpleCΔmucR1cells harbouring either themucR1-(3) ormucR1Tn5-plasmid (4). Molecular size standards are indicated on the left as blue lines with the corresponding values (blue) in kDa. (c,d) Occupancy of MucR1 (c) and MucR2 (d) at PpilAinWT, ΔpleC mucR1::Tn5double-mutant andmucR1::Tn5single-mutant cells as determined by qChIP using antibodies to MucR1 or MucR2. Data are from three biological replicates. Error is shown as s.d. (e) Immunoblots showing MucR1 and PilA steady-state levels inWT(a), ΔpleC(b), ΔpleC mucR1::Tn5double-mutant (c,d) and ΔpleCΔmucR1ΔmucR2(e) triple-mutant cells. ThemucR1::Tn5allele encodes a truncated derivative of MucR1. Molecular size standards are indicated on the left as blue lines with the corresponding values (blue) in kDa. (f) Immunoblots showing MucR2 and MreB (loading control) steady-state levels inWT(1), ΔmucR2(2),mucR1::Tn5(3) and ΔpleC mucR1::Tn5double-mutant (4) cells. Molecular size standards are indicated on the left as blue lines with the corresponding values (blue) in kDa. (g) Regulatory network showing putative promoters (dots) bound by CtrA, MucR1, MucR2 and SciP as inferred from ChIP-seq results inWTcells (Fig. 2). Common targets between MucR1 and MucR2 are shown in purple, between CtrA and SciP are shown in turquoise and between MucR and CtrA in red. This last group is subdivided into those bound by MucR1/MucR2/CtrA (a), MucR1/CtrA (b) and MucR2/CtrA (c). Note that MucR1/2 and SciP have few common targets. See alsoSupplementary Data 8for a prediction of specific and common MucR1 and MucR2 targets. (h). Scheme showing the predicted direct regulatory interactions at G1 or late S-phase promoters inferred fromg. Figure 3: Identification of mucR1/2 as negative regulator of PleC:CtrA promoters. ( a ) Growth of WT (a) Δ pleC (b) and derivatives (c,d) carrying the pilA :: P pilA –nptII transcriptional reporter on PYE plates containing kanamycin (20μg ml −1 ). ( b ) Immunoblot showing PilA steady-state levels in WT and Δ pleC Δ mucR1 double-mutant cells harbouring the empty vector (1 and 2, respectively), and Δ pleC Δ mucR1 cells harbouring either the mucR1- (3) or mucR1 Tn 5 -plasmid (4). Molecular size standards are indicated on the left as blue lines with the corresponding values (blue) in kDa. ( c , d ) Occupancy of MucR1 ( c ) and MucR2 ( d ) at P pilA in WT , Δ pleC mucR1 ::Tn 5 double-mutant and mucR1 ::Tn 5 single-mutant cells as determined by qChIP using antibodies to MucR1 or MucR2. Data are from three biological replicates. Error is shown as s.d. ( e ) Immunoblots showing MucR1 and PilA steady-state levels in WT (a), Δ pleC (b), Δ pleC mucR1 ::Tn 5 double-mutant (c,d) and Δ pleC Δ mucR1 Δ mucR2 (e) triple-mutant cells. The mucR1 ::Tn 5 allele encodes a truncated derivative of MucR1. Molecular size standards are indicated on the left as blue lines with the corresponding values (blue) in kDa. ( f ) Immunoblots showing MucR2 and MreB (loading control) steady-state levels in WT (1), Δ mucR2 (2), mucR1 ::Tn 5 (3) and Δ pleC mucR1 ::Tn 5 double-mutant (4) cells. Molecular size standards are indicated on the left as blue lines with the corresponding values (blue) in kDa. ( g ) Regulatory network showing putative promoters (dots) bound by CtrA, MucR1, MucR2 and SciP as inferred from ChIP-seq results in WT cells ( Fig. 2 ). Common targets between MucR1 and MucR2 are shown in purple, between CtrA and SciP are shown in turquoise and between MucR and CtrA in red. This last group is subdivided into those bound by MucR1/MucR2/CtrA (a), MucR1/CtrA (b) and MucR2/CtrA (c). Note that MucR1/2 and SciP have few common targets. See also Supplementary Data 8 for a prediction of specific and common MucR1 and MucR2 targets. ( h ). Scheme showing the predicted direct regulatory interactions at G1 or late S-phase promoters inferred from g . Full size image Unexpectedly, and in contrast to the mucR1 ::Tn 5 allele, an in-frame deletion of mucR1 (Δ mucR1 ) did not mitigate the defect in P sciP - lacZ and P pilA - lacZ transcription ( Fig. 1c and Supplementary Fig. 2A,B ) and PilA expression ( Fig. 3b ) of Δ pleC cells. However, when an in-frame deletion of mucR1 was introduced along with a deletion in the gene encoding the MucR2-paralog CC_0949 ( CCNA_00998 , henceforth mucR2, ), the P sciP - lacZ and P pilA - lacZ activity in the Δ pleC Δ mucR1/2 triple mutant even exceeded that of the Δ pleC mucR1 ::Tn 5 cells ( Supplementary Fig. 2A,B ). By contrast, reporter activity was hardly altered after deletion of either mucR1 or mucR2 from Δ pleC cells ( Supplementary Fig. 2A,B and Table 1 ). Table 1 Activity of MucR1/2-bound C. crescentus promoters in C. crescentus . Full size table Trans-dominance of mucR1 ::Tn 5 on mucR2 The results above suggest that the mucR1 ::Tn 5 insertion not only disrupts mucR1 but also causes trans -dominance on mucR2 . Several findings support this conclusion. First, a multi-copy plasmid carrying the coding sequence of truncated MucR1 from mucR1 ::Tn 5 (pMT335- mucR1 Tn 5 , see Methods section) alleviates the PilA ( Fig. 3b ) and P pilA - lacZ ( Supplementary Fig. 2C ) expression defect of Δ pleC Δ mucR1 double-mutant cells, while an analogous plasmid with WT mucR1 (pMT335- mucR1 ) does not. Second, MucR1 and MucR2 directly associate with P pilA and P sciP in vitro (as determined by electrophoretic mobility shift assays (EMSA); Supplementary Fig. 2D,E ) and in vivo (qChIP experiments conducted using polyclonal antibodies to MucR1 or to MucR2; Fig. 3c,d ). Third, mucR1 ::Tn 5 impairs binding of MucR2 at P pilA in vivo ( Fig. 3d ) and antibodies to MucR1 no longer precipitate P pilA from chromatin of mucR1 ::Tn 5 cells ( Fig. 3c ). As immunoblotting revealed that mucR1 ::Tn5 encodes a C-terminally truncated form of MucR1 ( Fig. 3e ) that does not affect MucR2 steady-state levels ( Fig. 3f ), we conclude that the mucR1 ::Tn 5 mutation not only removes codons required for DNA binding but also interferes with MucR2 binding to its targets. Finally, and most importantly, pull-down experiments using extracts of Δ mucR1 cells expressing a MucR1 derivative carrying C-terminal tandem affinity purification (TAP) tag revealed that MucR2 interacts with MucR1-TAP and MucR1 Tn 5 -TAP ( Fig. 4a ). 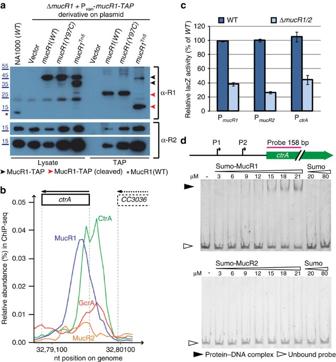Figure 4: Heterodimerization and auto-regulation by MucR1/2. (a) Immunoblots showing that MucR2 co-purifies with MucR1-TAP before (that is, in cell lysates, lysate) or after the first TAP purification step (cleavage with TEV protease, TAP). The upper panel shows a blot probed with antibodies to MucR1 (α-R1). The asterisk indicates untagged MucR1 in wild-type (NA1000) cells. The arrowheads indicate MucR1-TAP before (black) or after (red) cleavage of the protein-A moiety in the TAP tag with the TEV protease, eluting the proteins from the IgG agarose beads. The two lowest panels shows a blot probed with antibodies to MucR2 (α-R2) revealed at two different exposures. The lower amount of MucR2 that co-purifies withWTMucR1-TAP compared with MucR1(Y97C) or MucR1Tn5proteins is likely because of a reduction in the total MucR2 levels when MucR1 is overexpressed. Molecular size standards are indicated on the left as blue lines with the corresponding values (blue) in kDa. (b) Traces of the occupancy of various transcription factors at thectrApromoter based on ChIP-seq data. (c) β-Galactosidase measurements in extracts ofWT(dark blue) and ΔR1/2 (light blue) cells harbouring a PctrA-, PmucR1- or PmucR2-lacZpromoter-probe plasmid. Data are from three biological replicates. Error is shown as s.d. (d) Electrophoretic mobility shift assay (EMSA) showing the binding of His6-SUMO-MucR1 or -MucR2 to PctrA. The white arrows indicate the unbound probe. The black arrows indicate the shiftedctrAprobes bound by MucR1. His6-SUMO-MucR2 or His6-SUMO does not retard the probe. Figure 4: Heterodimerization and auto-regulation by MucR1/2. ( a ) Immunoblots showing that MucR2 co-purifies with MucR1-TAP before (that is, in cell lysates, lysate) or after the first TAP purification step (cleavage with TEV protease, TAP). The upper panel shows a blot probed with antibodies to MucR1 (α-R1). The asterisk indicates untagged MucR1 in wild-type (NA1000) cells. The arrowheads indicate MucR1-TAP before (black) or after (red) cleavage of the protein-A moiety in the TAP tag with the TEV protease, eluting the proteins from the IgG agarose beads. The two lowest panels shows a blot probed with antibodies to MucR2 (α-R2) revealed at two different exposures. The lower amount of MucR2 that co-purifies with WT MucR1-TAP compared with MucR1(Y97C) or MucR1 Tn 5 proteins is likely because of a reduction in the total MucR2 levels when MucR1 is overexpressed. Molecular size standards are indicated on the left as blue lines with the corresponding values (blue) in kDa. ( b ) Traces of the occupancy of various transcription factors at the ctrA promoter based on ChIP-seq data. ( c ) β-Galactosidase measurements in extracts of WT (dark blue) and Δ R1 /2 (light blue) cells harbouring a P ctrA -, P mucR1 - or P mucR2 - lacZ promoter-probe plasmid. Data are from three biological replicates. Error is shown as s.d. ( d ) Electrophoretic mobility shift assay (EMSA) showing the binding of His 6 -SUMO-MucR1 or -MucR2 to P ctrA . The white arrows indicate the unbound probe. The black arrows indicate the shifted ctrA probes bound by MucR1. His 6 -SUMO-MucR2 or His 6 -SUMO does not retard the probe. Full size image These findings along with the facts that MucR proteins can dimerize [24] , [27] and that eukaryotic zinc-finger transcriptional regulators form heterodimers [20] , [28] suggest that the trans -dominance of truncated MucR1 on MucR2 is due to the formation of inactive heterodimers. To map the residues in MucR1 that promote such trans -dominance on MucR2, we conducted random mutagenesis of mucR1 to isolate missense mutants that restore kanamycin resistance to Δ pleC pilA ::P pilA - nptII cells, akin to the mucR1 ::Tn 5 mutation. We isolated four mucR1 alleles encoding different single amino-acid substitutions (R85C, L87P, Y97C or Y97H; Supplementary Fig. 1D ; see Methods section) that disrupt one or both of the two conserved α-helices (residues 82-89 and 94-101) in the C-terminal DNA-binding domain of A. tumefaciens MucR/Ros determined by nuclear magnetic resonance spectroscopy (NMR) [24] . The residue corresponding to R85 of MucR1 is situated within the DNA recognition helix (helix 1) that along with basic residues in the N-terminal globular domain forms a surface-exposed patch that wraps around DNA and establishes specific base contacts [24] , suggesting that loss of this basic residue in MucR1 disturbs DNA binding. As pull-down assays showed that MucR1(Y97C)-TAP still interacts with MucR2 ( Fig. 4a ), we suggest that a MucR1(Y97C) homo-dimer and a MucR1(Y97C)-MucR2 heterodimer are non-functional, and that the other mutations are also loss-of-function mutations that can still interact with MucR2 and thus exert trans-dominance. Developmental control by MucR1 and MucR2 ChIP-seq analyses with antibodies to MucR1 and to MucR2 predicted 162 and 227 target sites for MucR1 and MucR2 ( Fig 2d,e ; and Supplementary Data 4 and 5 ), respectively. Cluster analyses of MucR1/2-, SciP- and CtrA target sites revealed a large overlap between CtrA, MucR1 and MucR2 targets (red set ‘a–c’, Fig. 3g ). Importantly, MucR1 and/or MucR2 bind G1-phase (PleC:CtrA) target promoters in vivo , but not SciP targets ( Supplementary Data 1 , as summarized in Fig. 3h ). The occupancy of CtrA and MucR1/2 over four selected promoter regions (including P pilA and P sciP ; Fig. 5a–d ) revealed overlapping or proximal peaks. Promoter-probe experiments with several of these target promoters confirmed their dependency on MucR1/2 in vivo ( Table 1 ). 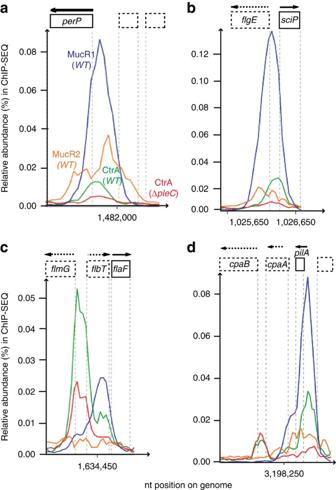Figure 5: PleC:CtrA target promoters that are bound and regulated by MucR1/2. (a–d) Traces of the occupancy of MucR1 (blue), MucR2 (orange) and CtrA (green) inWTcells and CtrA in ΔpleC(red) cells as determined by ChIP-seq data. Note that in panelc, the MucR1 binding overlaps the second binding site of CtrA upstream of theflaFgene. Figure 5: PleC:CtrA target promoters that are bound and regulated by MucR1/2. ( a – d ) Traces of the occupancy of MucR1 (blue), MucR2 (orange) and CtrA (green) in WT cells and CtrA in Δ pleC (red) cells as determined by ChIP-seq data. Note that in panel c , the MucR1 binding overlaps the second binding site of CtrA upstream of the flaF gene. Full size image In support of the notion that MucR1/2 regulates G1-phase promoters, simultaneous deletion of mucR1 and mucR2 from WT cells (Δ mucR1/2 ) imparts multiple developmental defects, disturbing the acquisition of motility, the buoyancy switch and holdfast gene expression (see below). These deficiencies are corrected when Δ mucR1/2 cells are complemented with a pMT335-derived plasmid harbouring mucR1 or mucR2 , but neither by a derivative harbouring mucR1 Tn 5 ( Fig. 6a,b ) nor by the distantly related mucR -paralog CC_1356 ( CCNA_01418 ). Moreover, the developmental defects are attenuated by mutations in ctrA or sciP that suppress the Δ mucR1/2 motility defect (see motile flare in Fig. 6b and Supplementary Fig. 3A,B ; see below). 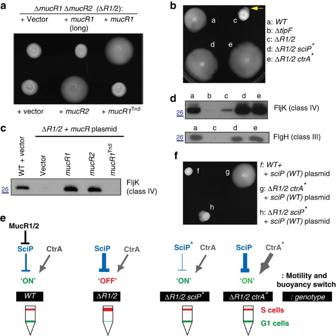Figure 6: Regulatory interplay betweenmucR1/2,sciPandctrAin the control of motility. (a,b). The motility defect of ΔmucR1ΔmucR2double-mutant cells (ΔR1/2)can be rescued by expression ofmucR1ormucR2from a plasmid or by point mutation insciPorctrA. (a) Motility plates (0.3% agar) inoculated with ΔR1/2cells containing the empty plasmid or derivatives withmucR1(long form, original annotation ofCC_0933),mucR1Tn5or the plasmids carryingmucR1(CCNA_00982) ormucR2 (CCNA_00998). (b) The motility of ΔR1/2(c) cells harbouring point mutation insciP(d) or inctrA(e) relative toWTcells (a). The yellow arrow points to the emergence of motile suppressors from a non-motile inoculum of ΔR1/2cells (c) versusWT(a) cells on motility agar. (c) Immunoblot showing the abundance of a class IV gene product (the FljK flagellin) in the supernatant ofWTand ΔR1/2cells containing the plasmids described ina. Molecular size standards are indicated on the left as blue lines with the corresponding values (blue) in kDa. (d) Immunoblots showing the steady-state levels of a class IV gene product (the FljK flagellin) and a class III gene product (the FlgH L-ring protein) inWT(a), ΔR1/2(c), ΔR1/2 sciP* (d) and ΔR1/2-ctrA* (e) cells. Also shown are the FljK levels in ΔtipFcells as a comparison (b). Molecular size standards are indicated on the left as blue lines with the corresponding values (blue) in kDa. (e) Model based on the regulatory interactions elucidated above. Misregulation ofsciPexpression in ΔR1/2impairs motility. A hypomorphic allele ofsciP(sciP*) or hypermorphic allele ofctrA(ctrA*) can restore motility to ΔR1/2cells. The buoyancy phenotype inWTand mutant cells is shown underneath. Note that thesciP* andctrA* mutations restore theWTbuoyancy phenotype, indicating adequate regulation of buoyancy effector(s). (f) ThesciPoverexpression plasmid pMT335-sciPinhibits motility in theWT(f) and in ΔR1/2 sciP* (h), but not ΔR1/2ctrA* (g) cells. Figure 6: Regulatory interplay between mucR1/2 , sciP and ctrA in the control of motility. ( a , b ). The motility defect of Δ mucR1 Δ mucR2 double-mutant cells (Δ R1/2) can be rescued by expression of mucR1 or mucR2 from a plasmid or by point mutation in sciP or ctrA . ( a ) Motility plates (0.3% agar) inoculated with Δ R1/2 cells containing the empty plasmid or derivatives with mucR1 (long form, original annotation of CC_0933 ), mucR1 Tn 5 or the plasmids carrying mucR1 ( CCNA_00982 ) or mucR2 (CCNA_00998) . ( b ) The motility of Δ R1/2 (c) cells harbouring point mutation in sciP (d) or in ctrA (e) relative to WT cells (a). The yellow arrow points to the emergence of motile suppressors from a non-motile inoculum of Δ R1/2 cells (c) versus WT (a) cells on motility agar. ( c ) Immunoblot showing the abundance of a class IV gene product (the FljK flagellin) in the supernatant of WT and Δ R1/2 cells containing the plasmids described in a . Molecular size standards are indicated on the left as blue lines with the corresponding values (blue) in kDa. ( d ) Immunoblots showing the steady-state levels of a class IV gene product (the FljK flagellin) and a class III gene product (the FlgH L-ring protein) in WT (a), Δ R1/2 (c), Δ R1/2 sciP * (d) and Δ R1/2 - ctrA * (e) cells. Also shown are the FljK levels in Δ tipF cells as a comparison (b). Molecular size standards are indicated on the left as blue lines with the corresponding values (blue) in kDa. ( e ) Model based on the regulatory interactions elucidated above. Misregulation of sciP expression in Δ R1/2 impairs motility. A hypomorphic allele of sciP ( sciP *) or hypermorphic allele of ctrA ( ctrA *) can restore motility to Δ R1/2 cells. The buoyancy phenotype in WT and mutant cells is shown underneath. Note that the sciP * and ctrA * mutations restore the WT buoyancy phenotype, indicating adequate regulation of buoyancy effector(s). ( f ) The sciP overexpression plasmid pMT335- sciP inhibits motility in the WT (f) and in Δ R1/2 sciP * (h), but not Δ R1/2 ctrA * (g) cells. Full size image The mucR1/2 - sciP-ctrA regulatory module Promoter-probe and immunoblotting experiments revealed that the activity of flagellar promoters ( Supplementary Fig. 3E ) and the abundance of class III and class IV flagellar proteins are diminished in Δ mucR1/2 cells relative to WT ( Fig 6c,d ). Since class II flagellar promoters are bound by SciP (but not MucR1/2, see above) in vivo and required for expression of class III and IV flagellar genes [14] and since transcription of sciP is negatively regulated by MucR1/2 ( Supplementary Fig. 2B ), we hypothesized that SciP represses S-phase promoters ectopically in Δ mucR1 /2 cells ( Fig. 6e ). Four lines of evidence support this conclusion. First, the promoters that are most efficiently bound by SciP in vivo ( Supplementary Data 2 , including P pleA , P flgB , P CC_3676 and P CC_3439 ) are the most downregulated in Δ mucR1 /2 cells ( Supplementary Figs 3E and 4A ). Second, as predicted, CtrA also targets these four promoters ( Supplementary Fig. 4 ) and induces a peak in transcript accumulation in S-phase [16] . Third, suppressor mutations in either sciP or ctrA augment the activity of these promoters in Δ mucR1 /2 cells ( Supplementary Fig. 4A ). Fourth, comparative ChIP-seq of WT and Δ mucR1 /2 cells revealed an increase in abundance of SciP at its preferred target sites in Δ mucR1 /2 versus WT cells (for example, with a log 2 difference of <−0.6 for P CC_3676 , P CC_3439 , P fliQ , P pleA , and P fliX ; Supplementary Data 6 ). Thus, while the mucR1/2-sciP-ctrA module maintains the correct balance in motility gene expression, deletion of mucR1/2 introduces an imbalance in regulation through SciP. The eleven suppressor mutations in sciP that we isolated are scattered throughout the entire (93-residue) coding region ( Supplementary Fig. 3B ), suggesting that reduced SciP function (or abundance) can be beneficial in the absence of MucR1/2. Importantly, the T65A mutation lies in a residue previously implicated in SciP function [17] , and we observed that derivatives of pMT335 harbouring either sciP(T24I) or sciP(T65A) are less efficient than the WT sciP version in inhibiting motility (of WT cells; Supplementary Fig. 3F ). The three suppressor mutations that we found in ctrA (encoding T168A, T170A and T170P; Supplementary Fig. 3A ) all map to the predicted DNA-binding domain. Interestingly, a related mutation (T170I) encoded by the ctrA401ts allele [12] impairs motility and prevents growth at 37 °C, while allowing growth at 28 °C. By contrast, WT strains harbouring ctrA(T170A) in place of WT ctrA exhibited no such temperature sensitivity. Thus, unlike the hypomorphic ctrA401ts allele, ctrA(T170A) acts as a hypermorphic allele. In support of this conclusion, motility is not inhibited upon mild overexpression of SciP from pMT335 in ctrA(T170A) cells. By contrast, ctrA + cells harbouring pMT335- sciP are non-motile ( Fig. 6f ; and Supplementary Fig. 3C,D ). These findings support the conclusion that transcription of sciP in G1-phase prevents activation of motility and other S-phase genes by CtrA ( Fig. 6e ), and that inappropriate expression of sciP from a multi-copy plasmid or by the Δ mucR1 /2 mutation prevents activation of these promoters in S-phase. Hypomorphic mutations in SciP (for example, T65A) or hypermorphic mutations in the CtrA DNA-binding domain (for example, T170A) mitigate these effects, presumably because the T170A substitution enhances CtrA’s ability to compete against repression by SciP in vivo . The Δ mucR1 /2 mutation also results in a diminished promoter activity (67% reduction versus WT ) of the hfsJ holdfast gene ( CC_0095 ) [29] and a buoyancy defect ( Fig. 6e ). Although the genetic basis of the Caulobacter buoyancy has not yet been determined, we found that the Δ mucR1 /2 buoyancy defect is reversed by the suppressor mutations in sciP and ctrA ( Fig. 6e ). Thus, the mucR1/2-sciP-ctrA module appears to act on an unknown buoyancy gene(s). Intriguingly, our ChIP-seq experiments revealed that the 26-kb genomic island that is located circa 480-kb clockwise from Cori and encodes at least one unknown buoyancy determinant [30] harbours the preferred binding sites of MucR1 and target sites of MucR2 ( Figs 2d–f ; and Supplementary Data 4,5 and 7 ). To explore this defect further, we conducted a himar1 transposon ( Tn ) mutagenesis experiment in mucR1/2 mutant cells and uncovered five buoyancy pseudo-reversion mutants, each harbouring a Tn insertions in the same gene ( CCNA_04006, encoded on the aforementioned 26-kb genomic island, Fig. 2f ) whose predicted translation product resembles the putative N-acetyl-L-fucosamine transferase WbuB from Escherichia coli [31] . An in-frame deletion in CCNA_04006 (Δ CCNA_04006 ) recapitulates the buoyancy pattern of the Tn mutation in either Δ mucR1/2 or WT cells ( Fig. 2g ) and is corrected when CCNA_04006 is expressed from a plasmid (pMT335- CCNA_04006 ), indicating that deletion of mucR1/2 affects CCNA_04006- dependent buoyancy switch. Direct and positive auto-regulation of mucR1/2 and ctrA Above we reported the functional and regulatory interactions between mucR1/2 - sciP and between mucR1/2 - ctrA. Interestingly, MucR1/2 bind P sciP and the ChIP-seq data traces in Fig. 4b indicate that MucR1 also binds the ctrA promoter. This notion was confirmed by EMSAs showing that His 6 -SUMO-MucR1, but not His 6 -SUMO-MucR2 or His 6 -SUMO, binds a ctrA promoter probe ( Fig. 4d ), albeit with somewhat lower affinity than the P pilA or P sciP probes ( Supplementary Fig. 2D,E ). Moreover, transcription from a ctrA promoter reporter plasmid (P ctrA - lacZ ) is reduced by 60% in Δ mucR1 /2 cells ( Fig. 4c ). Thus, MucR can also act positively on its target promoters as observed for other MucR proteins [25] , [32] , and a direct regulatory and functional relationship exists between mucR and ctrA . ChIP-seq also indicated a direct auto- and cross-regulatory relationship between MucR1 and MucR2 ( Supplementary Data 4 and 5 ). P mucR1 - lacZ and P mucR2 - lacZ promoter-probe reporters are reduced by 62% and 72%, respectively, in Δ mucR1 /2 cells relative to WT ( Fig. 4c ). Although the steady-state levels of MucR1 and MucR2 remain fairly constant during the cell cycle ( Supplementary Fig. 5A ) and MucR1 occupancy at P pilA in Δ pleC cells is near the occupancy seen in WT cells, we found that a Tn 5 insertion in the cell cycle kinase genes divJ or divL (that act in the PleC-signaling pathway [13] ) increases the occupancy of MucR1 at P pilA in Δ pleC cells ( Supplementary Fig. 5B ). This divJ- or divL -dependent increase of MucR binding is not because of diminished CtrA occupancy at P pilA , P tacA or P fliL ( Supplementary Fig. 6A–C ). Moreover, the recruitment of RNAP to P pilA ( Supplementary Fig. 6D ) and the production of PilA is restored ( Supplementary Fig. 1D in ref. 33 ). Finally, the abundance of CtrA~P is not reduced by these mutations in divJ and divL ( Supplementary Fig. 6E ). Thus, components of the cell cycle regulatory circuitry such as DivJ and DivL can modulate the occupancy of MucR1 on its targets. Conversely, MucR1 directly regulates expression of the master cell cycle regulator CtrA. Taken together, we conclude that mucR 1/2 is a critical component of an integrated and homeostatic (auto)regulatory module, mucR1/2 - ctrA - sciP, in which MucR not only engages in a double-negative regulation (MucR and SciP), but also in a double-positive one (MucR and CtrA) that likely helps reinforce and/or synchronize the molecular events underlying the S→G1 transcriptional switch. Pan-genomic ChIP-seq reveals conserved target regulation To investigate whether the link of MucR with the cell cycle circuitry has been maintained during evolution, we first assessed the extent of the functional conservation in the symbiont S. fredii NGR234 (henceforth S. fredii ) that also contains two mucR -like genes: a00320 on the symbiotic plasmid pNGR234a and c07580 on the chromosome. Both a00320 and c07580 can substitute for Caulobacter mucR1/2 in motility control ( Fig. 7a ), as is also the case for the unique mucR homologues encoded in the genomes of the animal pathogen B. suis and the plant pathogen A. tumefaciens ( Fig. 7a ), indicating that expression of sciP and the downstream motility target genes are sufficiently controlled by the heterologous MucR proteins to support motility. Because of this functional conservation, we asked if direct regulatory interactions were also maintained. To this end, we conducted pan-genomic ChIP-seq analyses using the antibodies to Caulobacter MucR1 and MucR2 to identify promoters bound by MucR-like proteins in S. fredii ( Fig. 7b ; Supplementary Fig. 7A ; and Supplementary Data 4 and 5 ). We then used these promoters to show the converse genetic dependency, that is, that these MucR-bound S. fredii promoters are regulated by Caulobacter mucR1/2 . Indeed, promoter-probe experiments with Caulobacter WT and Δ mucR1 /2 cells revealed that six S. fredii promoters are regulated negatively and two positively by MucR1/2 (out of 10 promoters tested; Table 2 ). 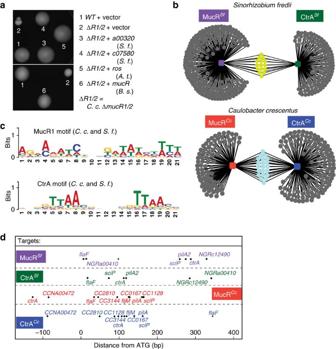Figure 7: Conservation of direct regulation by MucR and CtrA inC. crescentusandS. frediiNGR234. (a) Motility agar was inoculated withWTand ΔR1/2containing the empty vector or derivatives withmucRhomologues from different alpha-Proteobacteria:S. fredii (S. f) a00320(3) andS. f c07580(4),A. tumefaciens(A. t)ros(5),B. suis(B. s)mucR(6). (b) Network of DNA targets shared by CtrA and MucR inS. frediistr. NGR234 (S. f., upper) and inC. crescentus(C. c.,lower). (c)In silicodeduced binding motif of CtrA and MucR forC. c.andS. f. (d) Relative distance of CtrA- and MucR1-binding site relative to the ATG of common targets inC. c.and inS. f. NGR_c12490is orthologous toCC_0167andNGR_a00410toCCNA_00472. Figure 7: Conservation of direct regulation by MucR and CtrA in C. crescentus and S. fredii NGR234. ( a ) Motility agar was inoculated with WT and Δ R1/2 containing the empty vector or derivatives with mucR homologues from different alpha-Proteobacteria: S. fredii (S. f) a00320 (3) and S. f c07580 (4), A. tumefaciens ( A. t ) ros (5), B. suis ( B. s ) mucR (6). ( b ) Network of DNA targets shared by CtrA and MucR in S. fredii str. NGR234 ( S. f. , upper) and in C. crescentus ( C. c., lower). ( c ) In silico deduced binding motif of CtrA and MucR for C. c. and S. f . ( d ) Relative distance of CtrA- and MucR1-binding site relative to the ATG of common targets in C. c. and in S. f. NGR_c12490 is orthologous to CC_0167 and NGR_a00410 to CCNA_00472 . Full size image Table 2 Activity of MucR-bound S. fredii promoters in C. crescentus . Full size table Next, we attempted to compute pan-genomic consensus motif for MucR from the top 50 MucR1 target sites of Caulobacter and S. fredii ( Fig. 7c ) using the MEME algorithm (see Methods section). As proof-of-principle, we also computed a pan-genomic consensus motif of the top 50 CtrA-bound sites in the Caulobacter and S. fredii genomes determined by ChIP-seq using antibodies to Caulobacter CtrA ( Supplementary Data 7 ). The deduced motif is remarkably similar to the CtrA target sequence determined biochemically for Caulobacter (TTAA-N7-TTAA; Fig. 7c ), showing that this strategy can accurately predict consensus motifs. The pan-genomic consensus motif that was deduced for MucR1 is fairly degenerate, revealing a preference for AT-rich DNA substrates in GC-rich genomes (65% for Caulobacter and 61% for S. fredii ). Indeed, synthetic reporters (T5_ mucR1 b- lacZ and two attenuated derivatives; Supplementary Note 1 ) in which two MucR1 motifs were placed in tandem, downstream of a heterologous strong promoter from E. coli T5 phage driving lacZ expression are MucR-dependent in Caulobacter ( Supplementary Fig. 8A,B ), thereby validating our predicted pan-genomic MucR1-consensus sequence as a MucR1 target. Finally, we compared the target sites of CtrA and MucR in S. fredii using the consensus sequences. This revealed a suite of overlapping (or proximal) targets as for Caulobacter , albeit fewer in number ( Fig. 7b ). Importantly, several of these target sites in S. fredii are linked to orthologous genes that we determined to be under MucR and CtrA control in Caulobacter (including flaF - and sciP -like genes that are cell cycle-regulated and perform developmental functions in Caulobacter ; Fig. 7d ) [4] , [34] . Thus, the functional and direct regulatory relationships between MucR proteins and the cell cycle are (at least partly) conserved during evolution. Through forward genetics and (pan)genomic promoter occupancy of key cell cycle transcriptional regulators, we unearthed a conserved regulatory module, mucR1/2 - sciP-ctrA, that implements the S→G1 switch in Caulobacter . The ancestral zinc-finger transcription factor paralogs MucR1/2 repress G1-phase promoters that are activated by the essential master regulator CtrA including that controlling the negative regulator SciP that turns off S-phase promoters activated by CtrA. Through this double-negative wiring, the induction of G1-promoters occurs concomitantly with the repression of S-phase promoters. Superimposed on this double-negative regulatory wiring is a double-positive circuit in which MucR1/2 promotes expression of CtrA. Thus, MucR has both negative and positive roles in reinforcing the S→G1 transcriptional switch in Caulobacter . Remarkably, G1-phase-specific transcripts were recently also detected in synchronized S. meliloti [5] , raising the intriguing possibility that the underlying regulatory mechanisms that direct G1-phase transcription in Caulobacter also operate in symbiotic or virulent relatives, and that the mucR - sciP-ctrA regulatory module coordinates virulence/symbiosis and cell cycle transcription. Several findings are consistent with this notion. First, MucR proteins were previously described as regulators of virulence and symbiosis gene expression in Brucella , Sinorhizobia and Agrobacteria that also divide asymmetrically [3] , [25] , [35] . Second, we showed that MucR1/2 are required for proper implementation of the cell cycle transcriptional programs in dividing Caulobacter cells. Third, we found that MucR from Brucella , Sinorhizobia and Agrobacteria can confer motility to Caulobacter Δ mucR1 /2 mutants, a function that is dependent on proper cell cycle-dependent expression of SciP in G1-phase, while mis-expression of SciP impairs motility gene expression and leads to non-motile cells in soft agar ( Fig 6b,f ). Fourth, MucR-bound promoters of S. fredii NGR234 are also under MucR1/2 control in Caulobacter ( Table 2 ). Finally, our pan-genomic-binding site studies in Caulobacter and in the symbiont S. fredii revealed that many orthologous genes carry binding sites for MucR and CtrA in both species ( Fig. 7d ). With this close interplay of cell cycle transcription and virulence/symbiotic functions in mind, it is tempting to propose that certain transcriptional regulators previously thought to function exclusively as regulators of virulence/symbiosis should be re-classified as regulators of cell cycle transcription that restrict virulence gene expression to a specific cell cycle stage. For example, MucR proteins could endow a G1-phase-arrested daughter cell in Brucella , Sinorhizobia , Agrobacteria and likely other Alpha-proteobacteria with the necessary transcripts to establish virulence or symbiosis in the host. Indeed, motility and cell envelope-associated polysaccharides (responsible for the muc oid colony morphology) are both critical for virulence and known to be MucR controlled in Sinorhizobia and Brucella [3] , [25] , [35] . Interestingly, the fact that heterologous MucR proteins control cell cycle transcription indicates that they are properly regulated in Caulobacter , implying that MucR control is conserved in the Alpha-proteobacteria [6] . MucR1/2 protein levels remain relatively constant during the Caulobacter cell cycle, suggesting that MucR is regulated post-translationally. Indeed, the ability of heterologous MucR proteins to support function in another host is easier to reconcile with regulation by a small molecule that is produced by most Alpha-proteobacteria, rather than by a very promiscuous factor that must recognize the different MucR proteins. Several Alpha-proteobacteria including Caulobacter and S. fredii encode multiple MucR paralogs, and we show that the Caulobacter MucR paralogs can heterodimerize akin to eukaryotic zinc-finger transcription factors [28] . Although a single endogenous or a heterologous MucR paralog can support cell cycle transcription in Caulobacter , it is conceivable that heterodimerization serves to fine-tune MucR activity and cell cycle transcription. With the eukaryotic mitochondrion having descended from an Alpha-proteobacterium [21] and ancestral zinc-finger transcription factors being primarily represented in the Alpha-proteobacterial lineages, it is conceivable that these transcription factors originated in an Alpha-proteobacterium that had undergone a duplication of the mucR gene. Strains and growth conditions Caulobacter NA1000 (ref. 10 ) and derivatives were grown at 30 °C in PYE (peptone–yeast extract) or M2G (minimal glucose). S. fredii NGR234 (ref. 36 ) was grown at 30 °C in tryptone–yeast extract. E. coli S17-1 λ pir [37] and EC100D (Epicentre Technologies, Madison, WI) were grown at 37 °C in Luria broth. The E. coli mutator strain XL1 Red (Agilent Technologies Inc., Cedar Creek, TX) was grown at 30 °C in Luria broth. Motility assays, swarmer cell isolation, electroporations, biparental matings and bacteriophage ΦCr-30-mediated generalized transductions were performed as described [33] , [38] , [39] , [40] . Identification of mucR1 The mucR1 ::Tn 5 insertion was identified using a modification of the kanamycin resistance suppressor screen [33] . In brief, we screened for mini-Tn5 insertions that restore P pilA firing to Δ pleC cells bearing P pilA - nptII transcriptional reporter that confers kanamycin resistance to 20 μg ml −1 when P pilA is fully active. In contrast to previous screens that were done using a mini-Tn 5 conferring resistance to tetracycline, in this screen a version was used that confers resistance to gentamycin. The delivery plasmids pSS88 and pSS87 (ref. 41) [41] were used to mutagenize Δ pleC pilA :: P pilA - nptII cells by biparental mating with the mini-Tn 5 , screening for colonies that were resistant to gentamycin (1 μg ml −1 ), kanamycin (20 μg ml −1 ) and nalidixic acid (20 μg ml −1 , nalidixic acid is used to counter-select against the E. coli donor in biparental matings). This mutagenesis screen gave rise to one isolate (NR513) with the desired resistance profile. The Tn 5 insertion in NR513 was mapped to the uncharacterized CC_0933 gene at nucleotide (nt) position 1061847 of the C. crescentus NA1000 genome sequence ( Supplementary Fig. 1C ) using arbitrarily primed PCR [33] . Strain constructions The Δ mucR1 and Δ mucR2 marker-less single and double deletions were introduced into WT (NA1000) and Δ pleC [42] cells using the standard two-step recombination sucrose counter-selection procedure induced by the pNPTS138 derivatives. The resulting strains are the Δ mucR1 and Δ mucR2 single mutants, the Δ pleC Δ mucR1 , Δ pleC Δ mucR2 and Δ mucR1 Δ mucR2 double mutants, and the Δ pleC Δ mucR1 Δ mucR2 triple mutant. Deletions were confirmed by PCR using outside primers that do not hybridize within the mucR deletion alleles carried on pNPTS138. The mucR1 ::Tn 5 mutation (conferring gentamycin resistance and encoding a truncated MucR1 derivative that is dominant negative on MucR2) was transduced from strain NR513 (see below) into the WT (NA1000) and Δ pleC strains by ?Cr30-mediated generalized transduction, yielding strains in which endogenous mucR1 is replaced by mucR1 ::Tn 5. The P- lacZ transcriptional reporter strains were made by electroporation of the different plac290-based transcriptional reporter plasmids into WT (NA1000), Δ pleC , Δ mucR1 Δ mucR2 , Δ pleC Δ mucR1 Δ mucR2 , and the motile Δ mucR1 Δ mucR2 second-site suppressor mutants UG1277 (Δ mucR1 Δ mucR2 sciP T24I ) and UG1280 (Δ mucR1 Δ mucR2 ctrA T170A ). The pleC ::Tn 5 derivatives shown in Fig. 1f were made by generalized transduction of from SC1035 (ref. 43 ) into NA1000 or Δ ctrA :: Ω cells harbouring pSAL14 or pCTD14 (ref. 44 ). Isolation of phosphomimetic variants of ctrA , ctrA gof We identified ctrA gof alleles (gain of function, gof) by virtue of their ability to allow growth as sole copy of ctrA in a strain lacking the gene encoding the hybrid histidine kinase/phosphatase CckA ( cckA ) gene. To this end, the pMT464-ctrA plasmid was passaged through the E. coli mutator strain XL1 Red. The mutant library was subsequently electroporated into the Δ cckA ::Gent; ctrA ::Spc double-mutant strain carrying pCTD14 (pJS14- ctrAD51E conferring resistance to chloramphenicol) [45] and colonies that grew in the presence of kanamycin (20 μg ml −1 ) and 0.3% xylose were selected, as they were candidates in which pCTD14 had been displaced by a mutant pMT464- ctrA plasmid that can support growth in the absence of CckA (note that pCTD14 and pMT464 have the same origin of replication). The new ctrA gof alleles were sequenced, excised by cleavage with Nde I and Eco RI and cloned into pMT335 for further analysis in strains carrying the plac290-based P pilA - lacZ reporter plasmid. The mutant variants identified code for D8G, D8N, D51E, N53D or M99I. Note that the isolation of D51E, a known phosphomimetic allele [44] , validates the screen. Isolation of missense mutations in mucR1 To isolate missense mutations in mucR1 that phenocopy the mucR1 ::Tn 5 mutation, plasmid pMT375- mucR1 was mutated by passage through E. coli XL1 Red mutator strain (Agilent Technologies) on ampicillin. The mutagenized plasmid library was then electroporated into Δ pleC Δ mucR1 ; P pilA - nptII cells, selecting for resistance to tetracycline (1 μg ml −1 ) and kanamycin (20 μg ml −1 ). The new loss-of-function mutations that phenocopy the effect of mucR1 ::Tn 5 were excised by restriction with Nde I and Eco RI and cloned on pMT335 to assess their effects in strains carrying the plac290-based P pilA - lacZ promoter-probe plasmid. Motility suppressors of Δ mucR1 Δ mucR2 double-mutant cells Spontaneous mutations that suppress the motility defect of the Δ mucR1 Δ mucR2 double mutant appeared as ‘flares’ that emanated from the non-motile colony after approximately 4–5 days of incubation. After isolating 14 motile Δ mucR1 /2 suppressor mutants, two isolates (UG1277 and UG1278) were subjected to whole-genome sequencing and mutations in the sciP gene ( sciP T24I and sciP T65A , respectively) were found. In UG1277, the threonine codon (ACT) at position 24 in sciP is changed to one encoding isoleucine (ATT). In UG1278, the threonine codon (ACG) at position 65 in sciP is changed to one encoding alanine (GCG). Since SciP has been implicated in the regulation of CtrA, we sequenced sciP and ctrA in other suppressor mutants and found a mutation in strain UG1280 ( ctrA T170A ) in which the codon of threonine (ACC) at residue 170 was exchanged for one encoding alanine (GCC). To confirm that the mutations sciP T24I and ctrA T170A were responsible for the suppression of motility defect of the Δ mucR1 Δ mucR2 double mutant, we backcrossed each of the mutations into the Δ mucR1 Δ mucR2 strain. To this end, a pNPTS138 derivative (pNPTS138-hook, conferring kanamycin resistance) was integrated by homologous recombination nearby the sciP locus in UG1277. Next, ΦCr-30-mediated generalized transduction was used to transfer the mutant sciP allele from UG1277 into the Δ mucR1 Δ mucR2 mutant. Finally, the sucrose counter-selection procedure (see above) was used to select for stains that had lost pNPTS138-hook by homologous recombination. To backcross ctrA T170A from UG1280 into Δ mucR1 Δ mucR2 strain and the WT (NA1000) parent, the pNPTS138 derivative (pNPTS138- ctrA - ds ) was integrated nearby the ctrA locus of UG1280 by homologous recombination. ΦCr-30-mediated generalized transduction was used to transfer the mutant ctrA allele from UG1280 into the recipients by selecting for kanamycin resistance. Clones that have lost pNPTS138- ctrA - ds by homologous recombination were probed for kanamycin resistance (on PYE plates supplemented with kanamycin) and motility (on swarm agar plates) following sucrose counter-selection. PCR and sequencing was used to verify the integrity of the three mutants in each backcrossing experiment. Isolation of transposon insertions in CCNA_04006 Transposon ( himar1 ) mutagenesis of the Δ mucR1 Δ mucR2 strain was done using an E. coli λpir donor harbouring pHPV414 as described [46] . The mutant library was grown in PYE and then subjected to Percoll density gradient centrifugation, followed by enrichment for cells where the dense swarmer cells band is normally found. After repeated cycles of enrichment (growth in PYE followed by Percoll density gradient centrifugation), the band containing dense cells was extracted and single colonies were isolated on PYE plates. The transposon insertion sites in five clones were mapped as described [46] to nt 475241, 475633, 475659, 475789 and 476186 of the NA1000 genome sequence. Protein purification and antibody production For antibody production, His 6 -MucR1 or His6-SUMO-SciP(T24I) was expressed from pCWR350 and pUG97 in E. coli Rosetta (DE3)/pLysS (EMD Millipore, Billerica, MA), respectively, and purified the recombinant proteins purified under standard native conditions using Ni 2+ chelate chromatography. They were used to immunize New Zealand white rabbits (Josman LLC, Napa, CA). His 6 -SUMO-MucR2 was expressed from pUG12 in E. coli Rosetta (DE3)/pLysS and purified using Ni 2+ chelate chromatography in phosphate-buffered 8 M urea (Qiagen, Hilden, Germany). The protein was excised from a 15 % SDS polyacrylamide gel and used to immunize rabbits. For EMSAs, soluble His 6 -SUMO-MucR1, His 6 -SUMO-MucR2 or His 6 -SUMO was purified from E. coli Rosetta (DE3)/pLysS containing pUG30, pUG41 or pET28a-His 6 -SUMO, respectively, under native conditions using Ni 2+ chelate chromatography. In brief, cells were pelleted, resuspended in lysis buffer (20 mM Tris, 500 mM NaCl, 2 mM MgCl 2 , 50 mM L-glutamic acid, 50 mM L-arginine and 10 mM imidazole; pH 8.8) and lysed by three passages through a French pressure cell at 20,000 PSI. After centrifugation at 100,000 g the supernatant was loaded onto a 1 ml HisTrap column (GE Healthcare, Fairfield, CT) and eluted with a linear gradient using the same buffer containing 500 mM imidazole. Electrophoretic mobility shift assays His 6 -SUMO-MucR1, His 6 -SUMO-MucR2 or His 6 -SUMO were always freshly diluted into the binding buffer (25 mM Tris, 100 mM KCl, 5 mM MgCl2, 5 % glycerol and 0.05 % dodecyl maltoside, pH 7.5) to test the binding to the different Cy3-labelled DNA fragments. They were mixed with BSA (0.5 mg ml −1 BSA), sonicated salmon sperm DNA (0.05 mg ml −1 , Invitrogen Carlsbad, CA) and the Cy3-labelled DNA fragments (25 nM) in a total volume of 15 μl. The samples were incubated at room temperature for 10 min, then 5 μl 4 × loading dye (4 × binding buffer in 40% glycerol) was added, the samples separated on a 4% TBE polyacrylamide gel and the gel was scanned with a Typhoon FLA 7000 imager (GE Healthcare). Gel-purified 5′ Cy3-labelled PCR fragments (Macherey-Nagel, Bethlehem, PA) were used as probes. qChIP assays Mid-log phase cells were cross-linked in 10 mM sodium phosphate (pH 7.6) and 1% formaldehyde at room temperature for 10 min and on ice for 30 min thereafter, washed three times in phosphate-buffered saline (PBS) and lysed in a Ready-Lyse lysozyme solution (Epicentre Technologies) according to the manufacturer’s instructions. Lysates were sonicated (Sonifier Cell Disruptor B-30, Branson Sonic Power Co., Danbury, CT) on ice using 10 bursts of 20 s at output level 4.5 to shear DNA fragments to an average length of 0.3–0.5 kbp and cleared by centrifugation at 14,000 r.p.m. for 2 min at 4 °C. Lysates were normalized by protein content, diluted to 1 ml using ChIP buffer (0.01% SDS, 1.1% Triton X-100, 1.2 mM EDTA, 16.7 mM Tris-HCl (pH 8.1), 167 mM NaCl plus protease inhibitors (Roche, Switzerland) and pre-cleared with 80 μl of protein-A agarose (Roche) and 100 μg BSA. Ten percent of the supernatant was removed and used as total chromatin input DNA as described before [47] . Two microliters of polyclonal antibodies to CtrA [44] , SciP [17] , [18] (note that for ChIP experiments reported in Supplementary Data 6 , we used antibodies that we raised against His6-SUMO-SciP), FlbD [48] , RpoC (Neoclone, Madison, WI), MucR1 or MucR2 were added to the remains of the supernatant, incubated overnight at 4 °C with 80 μl of protein-A agarose beads pre-saturated with BSA, washed once with low salt buffer (0.1% SDS, 1% Triton X-100, 2 mM EDTA, 20 mM Tris-HCl (pH 8.1) and 150 mM NaCl), high salt buffer (0.1% SDS, 1% Triton X-100, 2 mM EDTA, 20 mM Tris-HCl (pH 8.1) and 500 mM NaCl) and LiCl buffer (0.25 M LiCl, 1% NP-40, 1% sodium deoxycholate, 1 mM EDTA and 10 mM Tris-HCl (pH 8.1)), and twice with TE buffer (10 mM Tris-HCl (pH 8.1) and 1 mM EDTA). The protein DNA complexes were eluted in 500 μl freshly prepared elution buffer (1% SDS and 0.1 M NaHCO3), supplemented with NaCl to a final concentration of 300 mM and incubated overnight at 65 °C to reverse the crosslinks. The samples were treated with 2 μg of Proteinase K for 2 h at 45 °C in 40 mM EDTA and 40 mM Tris-HCl (pH 6.5). DNA was extracted using phenol:chloroform:isoamyl alcohol (25:24:1), ethanol precipitated using 20 μg of glycogen as carrier and resuspended in 100 μl of water. For deep sequencing (ChIP-seq), total chromatin input DNA was not saved. To determine the specificity of MucR antibodies, samples were prepared and treated as for the ChIP, but after the washing steps the beads were resuspended in SDS loading buffer and boiled. Data are from three biological replicates. Pull-down of MucR2 with MucR1-TAP Overnight cultures were used to inoculate 80 ml of PYE (containing 50 μM vanillate to induce expression of MucR1-TAP proteins) and cells were grown to an OD 600 of 0.5–0.6. Sodium phosphate (pH 7.6) and formaldehyde were added to the cultures to a final concentration of 10 μM and 1%, respectively, and the cells were incubated for 10 min at room temperature followed by 30 min on ice. Cells were harvested by centrifugation (6500, rpm, 10 min at 4 °C) and washed twice in PBS. Cell pellets were resuspended in 900 μl of resuspension buffer (50 mM sodium phosphate, pH 7.4, 1 mM EDTA, 50 mM NaCl, 10 mM MgCl 2 , 0.5% n-Dodecyl-β-D-maltoside, 1 × protease inhibitors (Complete™ EDTA-free, Roche)) and lysed at room temperature for 15 min with a Ready-Lyse lysozyme solution (Epicentre Technologies). Cell lysates were sonicated (Bioruptor Pico, Diagenode) at 4 °C using 10 cycles of 30 s and cleared by centrifugation at a relative centrifugal force (r.c.f.) of 18,188 g for 2 min at 4 °C. The supernatant was incubated with IgG Sepharose beads (GE Healthcare Bio-Sciences, Sweden) for 2 h 30 min at 4 °C, washed six times with IPP150 buffer (10 mM Tris-HCl pH 8, 150 mM NaCl and 0.1% NP-40) and four times with TEV buffer (IPP150 buffer plus 0.5 mM EDTA and 1 mM DTT), and incubated overnight at 4 °C with TEV buffer containing 100 U ProTEV Plus protease (Promega) to release the tagged complex. The eluate was used for SDS-PAGE and immunoblotting. Real-time PCR Real-time PCR was performed using a Step-One Real-Time PCR system (Applied Biosystems, Foster City, CA) using 5% of each ChIP sample (5 μl), 12.5 μl of SYBR green PCR master mix (Quanta Biosciences, Gaithersburg, MD), 0.5 μl of primers (10 μM) and 6.5 μl of water per reaction. Standard curve generated from the cycle threshold ( C t ) value of the serially diluted chromatin input was used to calculate the percentage input value of each sample. Average values are from triplicate measurements done per culture. The final data was generated from three independent cultures. The DNA regions analysed by real-time PCR were from nucleotide −287 to −91 relative to the start codon of pilA , −313 to +32 of fliL , −226 to +30 of tacA and −191 to +14 of sciP . EMSA probe preparation The different promoter regions were amplified in a PCR using plasmids pJS70 (plac290-based P pilA-lacZ transcriptional fusion), pCC_0903-lac290 ( sciP ) or chromosomal DNA of NA1000 ( ctrA ) as templates and with 5′-Cy3-labelled oligonucleotides pilACy3fw and pilACy3rev, sciPCy3fw and sciPCy3rev, ctrACy3fwshort and ctrACy3revshort, or CtrACy3fwlong and CtrACy3revlong (see Supplementary Table 1 for sequences of oligonucleotides). The 5′-Cy3-labelled PCR fragments were gel purified (Macherey-Nagel). β-Galactosidase assays β-Galactosidase assays were performed at 30 °C as described earlier [40] . Fifty microlitres of cells at OD 660nm =0.1–0.6 were lysed with chloroform and mixed with 750 μl of Z buffer (60 mM Na 2 HPO 4 , 40 mM NaH 2 PO 4 , 10 mM KCl and 1 mM MgSO 4 heptahydrate). A quantity of 200 μl of ONPG (4 mg ml −1 o-nitrophenyl-β-D-galactopyranoside in 0.1 M KPO 4 pH 7.0) were added and the reaction timed. When a medium-yellow colour was developed, the reaction was stopped with 400 μl of 1 M Na 2 CO 3 . The OD 420nm of the supernatant was determined and the units were calculated with the equation: U= (OD 420nm × 1,000)/(OD 660nm × time (in min) × volume of culture (in ml). The assays were done in triplicates and normalization was done by conversion of the Miller Units (absolute values) of one arbitrarily chosen WT construct or WT background as reference, set to 100%. All absolute values were then converted to relative values, averaged and the error was determined by calculation of the s.d. Data are from three biological replicates. Antibodies used for immunoblotting and ChIP Polyvinylidenfluoride membranes (Merck Millipore Headquarters, Billerica, MA) were blocked with PBS, 0.05% Tween 20 and 5% dry milk for 1 h and then incubated for 1 h with the primary antibodies diluted in PBS, 0.05% Tween 20 and 5% dry milk. The different antisera were used at the following dilutions: anti-MucR1 (1:10,000), anti-MucR2 (1:10,000), anti-CtrA (1:10,000) [44] , anti-PilA (1:5,000) [49] , anti-FlgH (1:10,000) [50] , anti-MreB (1:10,000) [51] , anti-FljK (1:50,000) [52] . The membranes were washed four times for 5 min in PBS and incubated 1 h with the secondary antibody diluted in PBS, 0.05% Tween 20 and 5% dry milk. The membranes were finally washed again four times for 5 min in PBS and revealed with Immobilon Western Blotting Chemoluminescence HRP substrate (Merck Millipore Headquarters). Antibodies used for ChIP are to CtrA [44] , SciP [17] , [18] , FlbD [48] , RpoC (Neoclone) and MucR1 or MucR2. In vivo phosphorylation measurements In vivo P 32 labelling followed by immunoprecipitations (see Supplementary Fig. 1D in ref. 33 ) were done from cultures of a single colony of cells picked from a PYE agarose plate that was washed with M5G medium lacking phosphate and was grown overnight in M5G with 0.05 mM phosphate to an optical density of 0.3 at 660 nm (ref. 47 ). The strains used were as in Radhakrishnan et al. [33] One millilitre of culture was labelled for 4 min at 28 °C using 30 μCi of γ-[ 32 P]ATP. Following lysis, proteins were immunoprecipitated with 3 μl of antiserum to CtrA. The precipitates were resolved by SDS-PAGE, and [ 32 P]-labelled CtrA was quantified using a Storm 820 PhosphorImager and ImageQuant software version 4.0 (Molecular Dynamics) and were normalized to the relative cellular content as determined by immunoblotting of lysates. Data are from three biological replicates. Plasmid constructions, ChIP-seq and bioinformatics analyses Details are described in the Supplementary Methods . Accession codes : All ChIP-seq data was deposited in the GEO database under accession number GSE52849 . How to cite this article : Fumeaux, C. et al. Cell cycle transition from S-phase to G1 in Caulobacter is mediated by ancestral virulence regulators. Nat. Commun. 5:4081 doi: 10.1038/ncomms5081 (2014).